Enhancement ofAedes aegyptisusceptibility to dengue byWolbachiais not supported 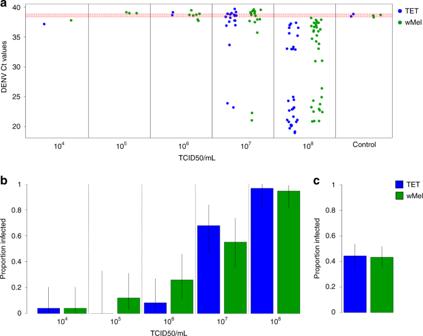Fig. 1: qPCR data and DENV infection rates from the original Souto-Maior et al.4data. aRaw DENV qPCR Ct values resulting from intrathoracic inoculations. Blue and green dots show Ct values from TET andwMel mosquitoes, respectively. Red dashed lines show Ct values from mock-injected negative controls.b–cProportions of TET andwMel mosquitoes classified by Souto-Maior et al.4(and likewise by King et al.3) as qPCR positive—proportions have been recalculated from the original dataset. Error bars show 95% binomial confidence intervals. 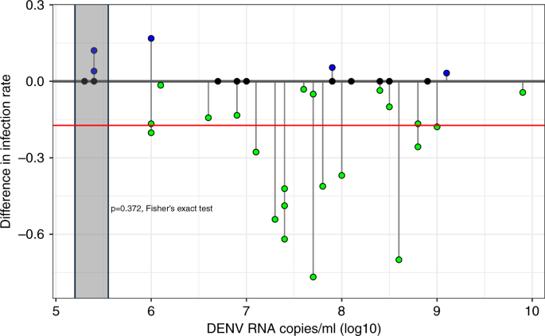Fig. 2: Differences in abdomen infection rate [(rate inwMel)—(rate inWolbachia-uninfected)] betweenwMel andWolbachia-negative mosquitoes fed on viremic blood, replotted from the original Ferguson et al.5data. Each dot represents a feeding on blood sourced from a different dengue-infected patient. Negative differences (green dots) indicate a lower abdomen infection rate inwMel-carrying mosquitoes. Positive differences (blue dots) indicate a higher abdomen infection rate inwMel-carrying mosquitoes. Black dots indicate no difference. The red line shows the mean difference across all DENV titres. Shaded area shows data points in the 105≤ X < 106RNA copies/ml stratum and statistical test. Further information on research design is available in the Nature Research Reporting Summary linked to this article.